The curved shape ofCaulobacter crescentusenhances surface colonization in flow Each bacterial species has a characteristic shape, but the benefits of specific morphologies remain largely unknown. To understand potential functions for cell shape, we focused on the curved bacterium Caulobacter crescentus . Paradoxically, C. crescentus curvature is robustly maintained in the wild but straight mutants have no known disadvantage in standard laboratory conditions. Here we demonstrate that cell curvature enhances C. crescentus surface colonization in flow. Imaging the formation of microcolonies at high spatial and temporal resolution indicates that flow causes curved cells to orient such that they arc over the surface, thereby decreasing the distance between the surface and polar adhesive pili, and orienting pili to face the surface. C. crescentus thus repurposes pilus retraction, typically used for surface motility, for surface attachment. The benefit provided by curvature is eliminated at high flow intensity, raising the possibility that diversity in curvature adapts related species for life in different flow environments. Bacteria have evolved a wide variety of morphologies [1] , but each species has a characteristic shape that is robustly maintained, indicating that specific shapes may provide bacteria with selective advantages in the wild. Much is known about the mechanisms by which bacteria acquire different shapes [2] , but what benefits do they confer? Despite numerous hypotheses, there remains no experimentally supported understanding of the advantages of specific morphologies [1] such as the curved shape of Caulobacter crescentus , a common model for studying bacterial cell cycle and polarity [3] . The curved morphology of C. crescentus requires the cytoskeletal protein crescentin (CreS), and any loss-of-function mutation in the creS gene results in straight rods [4] . Multiple independent natural C. crescentus isolates exhibit a similar ‘crescent’ shape [5] , indicating that cell curvature provides a selective advantage in the wild. However, in typical laboratory conditions, straight creS mutants maintain wild-type rates of growth and do not exhibit any obvious defect [4] . Given this paradox, we sought to identify what benefit C. crescentus might derive from its curved shape. C. crescentus is commonly found in freshwater lakes and streams [5] where surface colonization in the presence of fluid flow is a key determinant of fitness [6] , [7] . Multiple bacterial species have evolved the ability to form multicellular structures known as biofilms to robustly sustain growth in these environments. Similarly, C. crescentus populations grow as dense communities on surfaces in flow [8] , indicating that these cells must possess attachment mechanisms that promote local sessile colonization. To maintain surface attachment when subject to hydrodynamic forces, C. crescentus uses multiple adhesive structures [8] , including a strong adhesive holdfast at the tip of its polar stalk [9] , [10] , and pili and flagella that form at the opposite swarmer pole [11] . Given the apparent importance of surface attachment for C. crescentus , here we test the possibility that its curved shape plays a role in surface colonization in flow. Leveraging microfluidics to recreate the mechanical features of a natural environment that includes flow over a surface, we demonstrate that the curved shape of C. crescentus promotes surface colonization by enhancing the development of microcolonies that are larger and taller than those generated by straight mutants. We show that curvature improves surface colonization by bringing the piliated poles closer to the surface and orienting the pili towards the surface, thereby increasing the frequency of daughter cell attachment after division. We also demonstrate that crescent shape enhances microcolony spreading in the direction perpendicular to the flow, providing an explanation for how curvature enhances microcolony size and architecture. Finally, we provide evidence suggesting that C. crescentus leverages a single pilus retraction event seconds before daughter-cell separation to securely attach its progeny to the surface. These findings establish a mechanistic understanding of a possible benefit of bacterial curvature and provide new insights into the selective pressures that bacteria may encounter in their natural environments. Curved cells outcompete straight cells on surfaces in flow We grew C. crescentus in microchannels under steady flow and probed the effect of cell shape using time-lapse imaging to compare the growth of curved wild-type (WT) and straight creS cells ( Fig. 1a ). On growth in flow, and in contrast to growth in batch cultures, we found that curved cells have a pronounced advantage in surface colonization compared with straight cells. Specifically, in co-culture experiments with WT and creS mutants labelled with distinct fluorescent proteins, WT cells formed large and dense multicellular structures that we refer to as microcolonies ( Figs 1b , 2a,b and Supplementary Movies 1–4 ). WT cells formed wide, confluent microcolonies (green in Fig. 1b ) while creS mutants typically colonized the surface as isolated cells. Separately visualizing WT and creS on identical fluorescence intensity scales further revealed the significant advantage of WT during surface colonization ( Fig. 2a ). Relative to the creS mutant, WT cells exhibited an increased rate of colonization ( Fig. 2b,d , Supplementary Movies 1 and 2 ) and more microcolonies (in a 0.5 mm 2 area of the colonization surface, we detected 44 WT and 10 creS microcolonies after 20 h of growth). Confocal fluorescence microscopy also revealed that WT cells produced both wider and taller microcolonies ( Fig. 2c , Supplementary Movies 3 and 4 ). 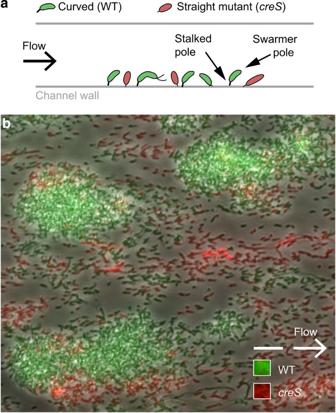Figure 1:C. crescentussurface colonization in flow. (a) Schematic of the competition experiments where curved (WT) and straight (creS)C. crescentusare initially attached to the microchannel surface. The channel depth is much larger than the dimensions of cells so that we can assume the top of the channel does not affect attachment. We apply pressure driven flow and observe microcolony formation or single-cell growth and division. (b) Overlay of phase and fluorescence images of a competition between WT CB15 (green) and straightcreS(red) cells after 32 h of growth under flow at the channel centerline. Scale bar is 10 μm. Swapping the fluorescent reporters yielded similar results (see Supplementary Fig 1 and Methods for details). In a separate control experiment without flow, there was no measurable difference in surface colonization, measured in arbitrary fluorescence units per hour, between WT (0.40±0.01 h −1 , mean±s.e.m.) and creS (0.39±0.02 h −1 ). In the absence of flow, neither WT nor creS formed clear microcolonies and the two populations co-colonized the surface uniformly at identical rates ( Fig. 3 ). We therefore attribute the surface colonization advantage of WT over creS to a coupling between cell shape and fluid flow. Figure 1: C. crescentus surface colonization in flow. ( a ) Schematic of the competition experiments where curved (WT) and straight ( creS ) C. crescentus are initially attached to the microchannel surface. The channel depth is much larger than the dimensions of cells so that we can assume the top of the channel does not affect attachment. We apply pressure driven flow and observe microcolony formation or single-cell growth and division. ( b ) Overlay of phase and fluorescence images of a competition between WT CB15 (green) and straight creS (red) cells after 32 h of growth under flow at the channel centerline. Scale bar is 10 μm. 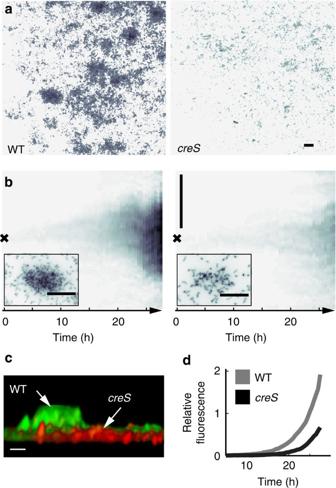Figure 2:C. crescentuscurvature enhances surface colonization. (a) Greyscale fluorescence images of comparing WT (left) andcreS(right) surface coverage after 20 h. (b) Spatial temporal plot of average fluorescence in the flow direction starting from a single WT (left) andcreS(right) cell. The insets show a snapshot of the colony at 24 h. The × signs at time zero indicate the position of the single cell that generated the colony. (c) Side (depth) view of adjacent WT andcreSmicrocolonies from confocal images after 24 h of growth. (d) Total fluorescent intensity as a function of time for the colonies shown inb. In all panels, we applied a flow generating a wall shear stress of 0.23 Pa at the channel centreline. Bar, 10 μm. Full size image Figure 2: C. crescentus curvature enhances surface colonization. ( a ) Greyscale fluorescence images of comparing WT (left) and creS (right) surface coverage after 20 h. ( b ) Spatial temporal plot of average fluorescence in the flow direction starting from a single WT (left) and creS (right) cell. The insets show a snapshot of the colony at 24 h. The × signs at time zero indicate the position of the single cell that generated the colony. ( c ) Side (depth) view of adjacent WT and creS microcolonies from confocal images after 24 h of growth. ( d ) Total fluorescent intensity as a function of time for the colonies shown in b . In all panels, we applied a flow generating a wall shear stress of 0.23 Pa at the channel centreline. Bar, 10 μm. 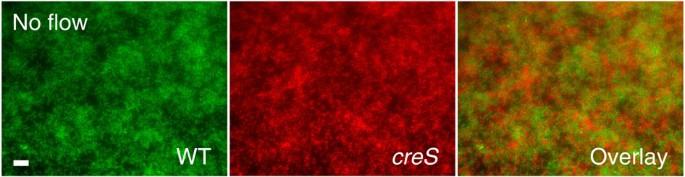Figure 3: Co-culture of WT andcreSmutant in the absence of flow. We show fluorescence images of WT (left, green),creS(middle, red) and their overlay (right) after 20 h. Curved and straight cells colonize the surface without forming the clear microcolonies observed in flow conditions. The measured rates of surface colonization show that WT does not have any significant growth advantage in the absence of flow. Scale bar is 10 μm. Full size image Figure 3: Co-culture of WT and creS mutant in the absence of flow. We show fluorescence images of WT (left, green), creS (middle, red) and their overlay (right) after 20 h. Curved and straight cells colonize the surface without forming the clear microcolonies observed in flow conditions. The measured rates of surface colonization show that WT does not have any significant growth advantage in the absence of flow. Scale bar is 10 μm. Full size image Curvature enhances daughter attachment in flow The dominance of curved cells in surface colonization under flow could be a result of a shorter doubling time or a higher rate of surface attachment. To distinguish between these possibilities, we compared WT and creS division in the presence of flow at single-cell resolution ( Fig. 4a , Supplementary Movie 5 ). We measured the average time between two daughter-cell separations and detected no statistically significant difference between their doubling times as WT divided in 85 min±1 min ( N =175) and creS in 84 min±1 min ( N =196) (Student’s t -test P -value=0.55). In contrast, tracking the fate of daughter cells after division revealed a significant difference in surface attachment probabilities for curved and straight cells. After each division, the stalked cell remains permanently attached to the surface, and the swarmer daughter cell, which does not initially harbour a holdfast, can either immediately reattach to the surface or be swept away by flow [12] . We calculated the probability of attachment ( p att ) as the ratio of swarmer cells that associated with the surface after division to the total number of observed divisions ( Fig. 4b ). On average, WT was twice as likely to attach ( p att =47%) than creS (24%). Thus, the curved shape of WT C. crescentus enhances the rate of surface colonization in the presence of flow by increasing the proportion of swarmer cells that attach to the surface. 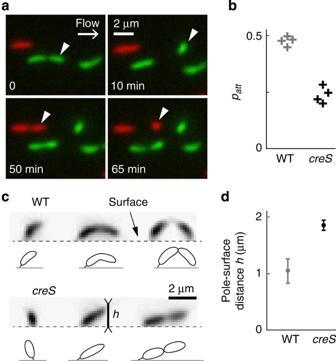Figure 4: Effect of cell curvature on swarmer cell attachment. (a) Fluorescence images of WT andcreScells dividing in flow. The top images show a WT swarmer initially attached to its mother (white arrowhead), which then separates and attaches to the surface 10 min later. The bottom images show a similar sequence for acreSswarmer (at 50 and 65 min). (b) Daughter-cell attachment probabilitiespattin four separate experiments (two for each fluorescent protein combination; sample sizes are provided inSupplementary Table 1). About one out of two WT daughter cells attach to the surface immediately after division while only one out of four does so forcreS. In the same experiments, we measured the time between two separations of daughter cell from a mother cell and measured statistically identical doubling times for WT (85 min±1 min, mean±s.e.m.,N=175) andcreS(84 min±1 min,N=196). (c) Cross-sectional views of WT andcreSgrowing in flow at different stages of the cell cycle with sketches of the basic shapes below. These reconstructions show distinct cells found at different stages of the life cycle. (d) Distancehfrom the surface to the swarmer pole of pre-divisional cells growing in flow. In these flow conditions, WT cells are in average 1 μm away from the surface whilecreSgrow at about 2 μm. The error bars show the 95% confidence intervals. In all panels, the applied flow generates a wall shear stress of 0.23 Pa. Figure 4: Effect of cell curvature on swarmer cell attachment. ( a ) Fluorescence images of WT and creS cells dividing in flow. The top images show a WT swarmer initially attached to its mother (white arrowhead), which then separates and attaches to the surface 10 min later. The bottom images show a similar sequence for a creS swarmer (at 50 and 65 min). ( b ) Daughter-cell attachment probabilities p att in four separate experiments (two for each fluorescent protein combination; sample sizes are provided in Supplementary Table 1 ). About one out of two WT daughter cells attach to the surface immediately after division while only one out of four does so for creS . In the same experiments, we measured the time between two separations of daughter cell from a mother cell and measured statistically identical doubling times for WT (85 min±1 min, mean±s.e.m., N =175) and creS (84 min±1 min, N =196). ( c ) Cross-sectional views of WT and creS growing in flow at different stages of the cell cycle with sketches of the basic shapes below. These reconstructions show distinct cells found at different stages of the life cycle. ( d ) Distance h from the surface to the swarmer pole of pre-divisional cells growing in flow. In these flow conditions, WT cells are in average 1 μm away from the surface while creS grow at about 2 μm. The error bars show the 95% confidence intervals. In all panels, the applied flow generates a wall shear stress of 0.23 Pa. Full size image We also measured the attachment probabilities of WT and creS in the absence of flow ( Supplementary Table 1 ). For both curved and straight cells, absence of flow reduced attachment compared with growth under flow. However, we still measured a higher attachment probability for WT ( p att =30%) over creS ( p att =16%), despite the lack of a surface colonization advantage for WT. To reconcile the observations that in the absence of flow WT cells have improved local attachment but no surface colonization advantage, we suggest that in the closed system resulting from the absence of flow the unattached cells are free to swim away and attach to the surface at a later time, thereby eliminating any net colonization advantage. This delayed and delocalized attachment could explain why densely packed microcolonies are not observed in the absence of flow. By contrast, the presence of flow causes unattached cells to be swept away out of the system, thereby generating a net colonization advantage for those cells that can locally attach before being caught up in the flow. How could a curved cell shape enhance local surface attachment? We visualized cell position in flow in three dimensions using deconvolution of fluorescence images ( Fig. 4c ). On initial attachment, both WT and creS mutants appeared to stand straight up (approximately perpendicular to the channel surface, Fig. 4c , left). As these cells and their stalks grew, WT and creS cells reoriented in the direction of flow in different manners. The curved WT cells formed an arc such that their swarmer pole was oriented towards the surface. As these cells grow in length, cell curvature causes the WT swarmer poles to bend towards the surface, such that the swarmer pole adhesins both point towards and get nearer to the surface ( Fig. 4c , middle). We found many cases of WT cells where both poles were simultaneously in contact with the substrate before cell separation is complete ( Fig. 4c , right). In contrast, as straight creS cells increase in length, the swarmer pole remains oriented away from the surface and constantly gets further away from the surface ( Fig. 4c , bottom). In these conditions, we found no cases of creS cells where both poles were simultaneously in contact with the surface ( Fig. 4c , bottom). Thus, cell shape may enhance surface attachment by spacing and orienting the cell pole relative to the surface during division. To provide quantitative support for our model that curvature in flow yields a geometrical advantage that promotes surface attachment, we measured the distance between the swarmer pole and the surface of pre-divisional cells. We reconstructed side views of visibly dividing cells using fluorescence z-stacks as in Fig. 4c and measured the distance h separating the swarmer pole from the surface that we report in Fig. 4d . Consistent with our hypothesis and the qualitative results of Fig. 4c , the distance between the swarmer pole and the surface was significantly shorter for curved WT cells ( h =1.0 μm±0.1 μm) than for straight creS cells ( h =1.8 μm±0.05 μm, Student’s t -test P -value <10 −3 ). These measurements further validate the hypothesis that the curved shape of C. crescentus enhances surface colonization by increasing the probability that swarmer pole adhesins interact with the surface. We note that our hypothesis also explains why WT cells attach better in the absence of flow, as curvature reduces the distance between the swarmer pole and the surface even when cells are oriented perpendicular to the surface. Orientation of an attached curved rod in flow When attached to a surface with its holdfast, a C. crescentus cell experiences a hydrodynamic force acting on its body and a spring-like force generated by its holdfast. The former tends to align the cell with the direction of flow while the latter opposes changes in orientation with respect to a rest position. To rationalize the physical mechanism by which flow enhances surface attachment of WT cells, we modelled C. crescentus as a curved rod to predict qualitatively its orientation as shown in Fig. 5 . For simplicity, we initially neglect the elastic force generated by the holdfast and assume that the cell is only free to rotate around the axis perpendicular to the surface (it remains in a vertical orientation) as in Fig. 5a . Because the cell is curved, viscous forces generate a torque that rotates the cell around the vertical axis so that the cell reorients in the direction of the flow. Under these assumptions, a cell that aligns with flow is in a stable conformation when oriented downstream: viscous forces restore this orientation on small perturbations, for example, when disturbed by Brownian effects. Conversely, the upstream orientation is unstable as illustrated in Fig. 5a . 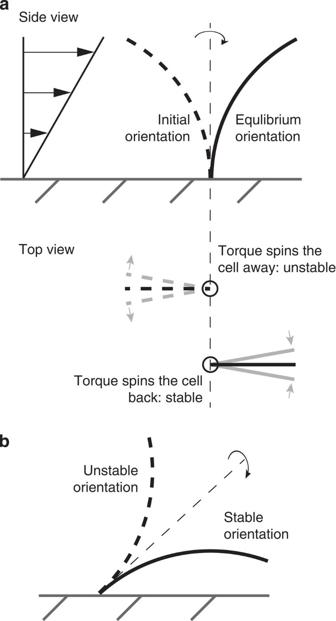Figure 5: Orientation of an attached curved-rod in flow. Ina, a vertical cell (attached via a holdfast and a stalk oriented vertically) experiences a torque generated by off-axis viscous forces applied on the curved body. The curved rod rotates about its vertical axis to reach a stable position, where the free pole points downstream. Upstream orientation is an unstable conformation as small perturbations lead viscous forces to generate a torque spinning the cell away from its initial position (top view). (b) A curved rod lying at an angle experiences similar torques, now generated by the velocity component perpendicular to the rotation axis. Similarly, the unique stable orientation is when the cell faces the surface. Figure 5: Orientation of an attached curved-rod in flow. In a , a vertical cell (attached via a holdfast and a stalk oriented vertically) experiences a torque generated by off-axis viscous forces applied on the curved body. The curved rod rotates about its vertical axis to reach a stable position, where the free pole points downstream. Upstream orientation is an unstable conformation as small perturbations lead viscous forces to generate a torque spinning the cell away from its initial position (top view). ( b ) A curved rod lying at an angle experiences similar torques, now generated by the velocity component perpendicular to the rotation axis. Similarly, the unique stable orientation is when the cell faces the surface. Full size image We now relax the assumption of the cell remaining in a vertical orientation, so that its body is free to orient at an angle with the vertical axis (as in Fig. 5b ). Qualitatively, the stability of each conformation is similar to the discussion above: the position where the cell pole is oriented downstream is stable, whereas the upstream orientation is unstable. Therefore, we predict that the cell will generally remain with its swarmer pole oriented downstream, that is, towards the surface. We note that, despite the cell being in a stable orientation with respect to the axis of its stalk, it is still subject to a torque generated by shear stress that tends to flip the cell in the direction of flow, similar to an ellipsoid describing a Jeffery orbit [13] . This effect is likely attenuated by an opposite torque exerted by the holdfast, wall effects, and the finite width of the cell that limits the accessible angles of orientation. We calculated the distance from the swarmer pole to the surface for similarly oriented curved and straight cells with typical dimensions and found that the swarmer pole of a curved cell is always closer to the surface than the pole of a straight cell ( Supplementary Fig. 5 ). The benefit in the angle of orientation of the pole to the surface scales linearly with cell length and is to the advantage of curved cells. To summarize, cell curvature in flow orients the curved cell in a stable orientation where its swarmer pole faces the surface, which allows for enhanced attachment of a daughter cell in flow. Flow intensity modulates the advantage in surface attachment To verify that the attachment probability of creS depends on the distance between their swarmer poles and the surface, we modulated this distance by controlling flow speed and measuring p att . Higher flow speeds should have little effect on the arced orientation of WT cells, but should cause straight cells to grow at a shallower angle relative to the surface, thereby decreasing the distance from the swarmer pole to the surface. In support of our hypothesis, we found that increasing the flow rate had little effect on the attachment probability of WT cells, while the attachment probability of creS mutants increased as a function of wall shear stress ( Fig. 6a and Supplementary Fig. 2 ). At higher flow speeds (wall shear stress larger than 2 Pa), the attachment probabilities of WT and creS mutants are nearly the same ( Fig. 6a ). In this regime, the swarmer poles of curved and straight cells are approximately at the same distance h from the surface ( Supplementary Fig. 3 ). Importantly, this result suggests that the intrinsic ability of WT and creS to attach is similar. Consequently, we can attribute the improved WT attachment at lower shear stress to the effect of cell shape on the orientation and position of the swarmer pole, rather than secondary effects on the quality of attachment. 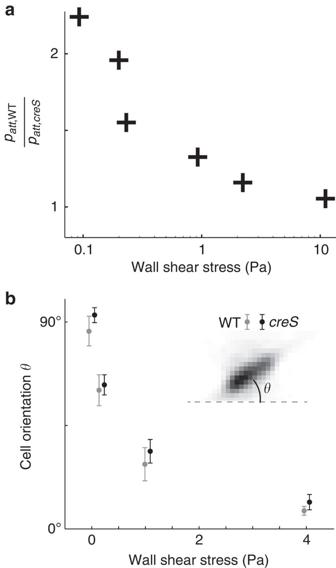Figure 6: Flow intensity modulates the attachment advantage by orienting cells. (a) Effect of increase in wall shear stress on the relative attachment probabilities (patt) of WT andcreSdaughter cells. (b) Cell body orientation as a function of wall shear stress. At zero flow, both WT (gray bars) andcreS(black bars) are standing up on the surface (θ=90°). At low flow, both WT andcreSorient towards the surface. They lay nearly parallel to the surface at wall shear stress above 4 Pa. The error bars show the 95% confidence intervals (N>50). Figure 6: Flow intensity modulates the attachment advantage by orienting cells. ( a ) Effect of increase in wall shear stress on the relative attachment probabilities ( p att ) of WT and creS daughter cells. ( b ) Cell body orientation as a function of wall shear stress. At zero flow, both WT (gray bars) and creS (black bars) are standing up on the surface ( θ =90°). At low flow, both WT and creS orient towards the surface. They lay nearly parallel to the surface at wall shear stress above 4 Pa. The error bars show the 95% confidence intervals ( N >50). Full size image We speculated that flow intensity could affect attachment by orienting the stalked cells with respect to the surface. We thus measured the angle between the channel surface and the cell as a function of flow intensity and correlated these values with swarmer cell attachment probability ( Fig. 6b ). At zero flow, both WT and creS cells are nearly perpendicular to the surface (θ≈90°). As predicted by our model, at intermediate flows (wall shear stress below 2 Pa), cells form a shallower angle with the surface as hydrodynamic forces overcome the elasticity of the holdfast. Further increasing the wall shear stress pushes the cell down against the channel wall, orienting its body nearly horizontally, parallel to the surface (θ≈10° at 4 Pa). These measurements of orientation further support our model that attachment probability increases when the distance from the swarmer pole to the surface h decreases. We calculated the distance h by projecting the cell body using typical cell dimensions (see Methods section). Supplementary Fig. 4 shows the negative correlation between p att and the distance h for both WT and creS . To further validate our model, we determined the shear stress at which WT and creS would be predicted to have identical attachment probabilities based on the distance of their pole to the surface (see Supplementary Discussion ). From our measurement of attachment probabilities and orientation, we predict that the two strains should have identical attachment probabilities when they are parallel to the surface (θ≈0°). By balancing the torque generated by the elasticity of the holdfast [14] with the torque generated by hydrodynamic forces, we predict that WT and creS would have similar attachment probabilities for a wall shear stress on the order of 10 Pa. This value is consistent with our experimental measurements of the shear stress where attachment probabilities for WT and creS converged to the approximately equal values value. Curvature spreads daughter cells transversely to the flow Curvature enhances expansion of WT microcolonies transverse to the direction of flow ( Figs 1b and 2b ) so that they grow into strikingly wider structures than straight cells. To test whether this is a consequence of faster microcolony growth or a feature of cell shape, we quantified the positions at which WT and creS swarmer cells attach to the surface after separation relative to their mother. With respect to the flow axis, we measured the axial and transverse distances between the stalked pole of each mother cell and the newly attached pole of its daughters ( Fig. 7a ). Most creS cells attach immediately downstream of their mother, as indicated by a narrow probability density. Conversely, WT cells spread significantly further away from the mother cell in the transverse direction. We used the s.d. of the transverse (vertical) coordinates of daughter cells to measure the extent of their dispersal. The daughter-cell distribution for WT spreads 2.8 μm transverse to the direction of the flow, compared with 1.6 μm for the creS mutant. This enhanced transverse spreading propagates with each division event, causing a single curved mother cell to produce a far broader microcolony than that produced by a straight cell ( Fig. 7b ). This likely leads to a broader and denser cell monolayer, allowing for development of a more robust three-dimensional biofilm architecture. 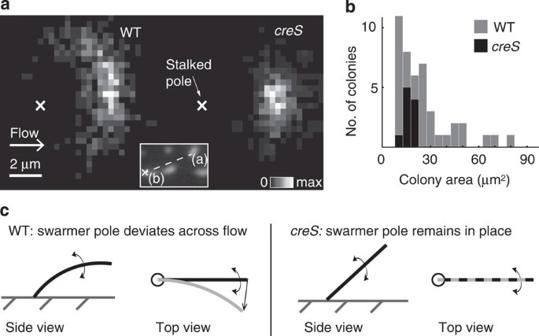Figure 7: Cell curvature enhances dispersal across flow to form larger microcolonies. (a) Probability density of attachment locations of daughter cells relative to the stalked pole of their mother. The inset shows the location of a swarmer daughter (a) relative to the stalked pole of its mother cell (b). (b) Histogram of area of contiguous cells from fluorescence in a 0.5 mm2area for WT andcreSmicrocolonies. The mean colony size is 26 μm2for WT and 17 μm2forcreS. (c) Side and top views of curved and straight rods with slight deviations from equilibrium position, aligned with flow and facing the surface, and of a curved rod aligned with flow slightly rotated about its axis (grey line). The slight rotation of the curved rod displaces the swarmer pole sideways, transverse to the direction of the flow. Therefore, any rotation of the cell axis disperses daughter cells transversally. Conversely, a straight cell is axis symmetric, so that any rotation about its axis leaves the swarmer pole in place. Figure 7: Cell curvature enhances dispersal across flow to form larger microcolonies. ( a ) Probability density of attachment locations of daughter cells relative to the stalked pole of their mother. The inset shows the location of a swarmer daughter (a) relative to the stalked pole of its mother cell (b). ( b ) Histogram of area of contiguous cells from fluorescence in a 0.5 mm 2 area for WT and creS microcolonies. The mean colony size is 26 μm 2 for WT and 17 μm 2 for creS . ( c ) Side and top views of curved and straight rods with slight deviations from equilibrium position, aligned with flow and facing the surface, and of a curved rod aligned with flow slightly rotated about its axis (grey line). The slight rotation of the curved rod displaces the swarmer pole sideways, transverse to the direction of the flow. Therefore, any rotation of the cell axis disperses daughter cells transversally. Conversely, a straight cell is axis symmetric, so that any rotation about its axis leaves the swarmer pole in place. Full size image We identified several features of curvature that could promote dispersal transverse to the flow. In flow, newly divided curved daughter cells reorient towards an equilibrium position ( Fig. 5 ), where hydrodynamic forces and torques on the cell body are balanced by those exerted by the holdfast. For a curved cell, any rotation about the axis away from its equilibrium position displaces the swarmer pole in a direction transverse to the flow ( Fig. 7c ), whereas the swarmer pole of a straight cell remains in place. Therefore, any factors causing cell body rotation, such as Brownian motion, local crowding or flagellar rotation, would cause transverse spreading of curved cells. These factors would also cause straight cells to rotate about their axis, but such rotation would leave the cell pole in place and thus not increase transverse dispersal. Thus, curved cell shape can rationalize both the increased local attachment and the increased microcolony formation observed for WT cells. Type IV pili mediates swarmer pole attachment Our results indicate that the combination of flow and cell curvature causes the swarmer cell pole to orient towards the surface, driving surface colonization. We hypothesized that orienting the swarmer pole towards the surface improves the ability of swarmer pole structures, flagella or type IV pili, to interact with the surface. We thus measured surface attachment probabilities for mutants lacking flagella ( flgE ) or type IV pili ( pilA ). While the flagellum-less cells remained efficient at attaching, the loss of pili eliminated the majority of attachment events for both WT and creS ( Supplementary Table 1 ). Further support for the role of swarmer-localized pili in surface attachment came from high-speed imaging of division. A few seconds before cell separation, WT swarmer poles often exhibited a sudden jerk of motion ( Fig. 8a and Supplementary Movie 6 ) similar to retraction events driven by pilus depolymerization [15] . We still observed these retraction-like events in mutants lacking flagella (clear retractions were observed in 15 out of 27 observed attachment events), but not in mutants lacking pili (0 out of 14 observed events). Type IV pili are more generally associated with twitching-based surface motility [16] , but C. crescentus does not twitch [17] . We propose that C. crescentus has re-purposed pili as retractable adhesins for surface attachment, consistent with previous work suggesting that C. crescentus pili retract only once per cell cycle near the time of division [18] , [19] . These studies of C. crescentus pilus development suggested that pili become functional after division. However, the low temporal resolution and assay methods of those studies made it impossible to distinguish whether pili become functional shortly before or after division. Our high-resolution time-lapse visualization sheds light on this question and indicates that C. crescentus pili can retract before mother and daughter cells separate. 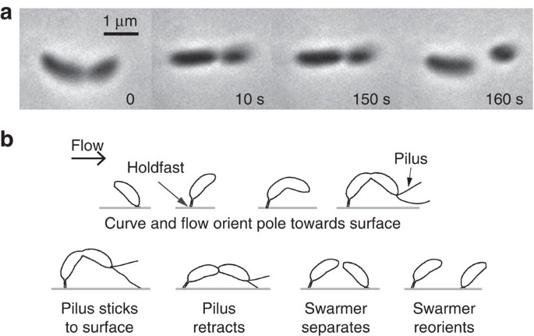Figure 8: Pilus retraction helps daughter cells attach to the surface before separation. (a) Phase contrast images of a separating swarmer cell. Initially, the dividing cell is attached. At 10 s, the swarmer pole rapidly moves towards the surface. The cell maintains this conformation before fully separating (160 s). (b) Model for the effect of cell shape on attachment during division. As an initially attached stalked cell grows in length, flow and cell curvature cause the cell to arc, orienting the piliated pole towards the surface and bringing it closer to the surface. This geometry increases the probability that pili will bind the surface, causing the swarmer daughter to remain surface attached after division rather than being swept away by the flow. Figure 8: Pilus retraction helps daughter cells attach to the surface before separation. ( a ) Phase contrast images of a separating swarmer cell. Initially, the dividing cell is attached. At 10 s, the swarmer pole rapidly moves towards the surface. The cell maintains this conformation before fully separating (160 s). ( b ) Model for the effect of cell shape on attachment during division. As an initially attached stalked cell grows in length, flow and cell curvature cause the cell to arc, orienting the piliated pole towards the surface and bringing it closer to the surface. This geometry increases the probability that pili will bind the surface, causing the swarmer daughter to remain surface attached after division rather than being swept away by the flow. Full size image Our results suggest a model for C. crescentus attachment in flow, which we illustrate in Fig. 8b . Initially, a curved C. crescentus cell irreversibly attaches to a surface with its holdfast. Fluid flow tends to orient the cell in the direction of flow, with the swarmer pole facing the surface. In this configuration, as the cell grows in length, curvature allows for a reduction of the distance between the surface and the swarmer pole. As it initiates division, the daughter cell synthesizes a flagellum (omitted in Fig. 8b ) and type IV pili at the swarmer pole. Through optimized orientation and reduced distance, curvature increases the probability for a pilus to encounter the surface. If pilus attachment is successful, pilus retraction allows for contact of the swarmer pole to the surface. The newly attached swarmer cell then fully separates from the stalked mother cell and can reorient while initiating division. Small perturbations in orientation increase dispersal in the transverse direction, allowing for the development of wider multicellular structures. In the absence of flow, curved cells lose their fitness advantage over straight cells as both populations uniformly colonize the surface at identical rates. In these conditions, WT daughter cells still maintain a higher probability of local attachment after division than creS . However, cells that do not attach at the time of division are not transported by flow. As a result, these planktonic cells will still attach to the surface at a later time. Given that WT and creS have identical doubling times, growth rates remain equal in this closed system, and therefore WT does not display a growth advantage, just as in a test tube. Consequently, shape is critical to the local attachment probability of newborn daughter cells, which specifically provides a surface colonization advantage in the presence of flow. Unlike other piliated bacteria that use successive rounds of pilus extensions and retractions as a surface motility mechanism [16] , C. crescentus pili retract only once per cell cycle at the time of division [18] . The timing of retraction (before cell separation) demonstrates the importance of the rapid attachment of daughter cells to the establishment of a surface-associated community. On contact, the transiently attached daughter cell disables flagellum rotation and initiates irreversible surface attachment by synthesizing a holdfast [9] . If pilus attachment is not successful, flow disperses the swarmer cell, which can immediately use its flagellum to swim in the bulk fluid to another environment as illustrated in Fig. 9 . 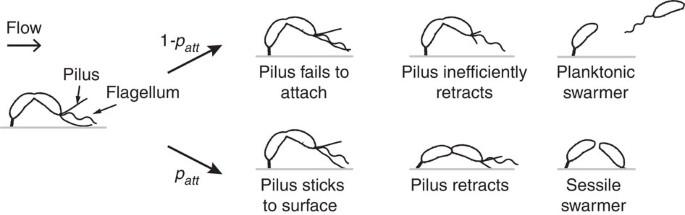Figure 9: Model illustrating the fate of daughter cells after division from an attached mother cell. After division, the daughter cell will either remain attached to the surface and live a sessile lifestyle (with probabilitypatt) or be released in the bulk of the fluid (with probability 1-patt). Dividing swarmers increase their chance of successful attachment by sticking a pilus on the surface followed by retraction before separation. Failure to stick a pilus leads to a release of the swarmer daughter in the bulk, where it is free to swim or be carried by flow. Figure 9: Model illustrating the fate of daughter cells after division from an attached mother cell. After division, the daughter cell will either remain attached to the surface and live a sessile lifestyle (with probability p att ) or be released in the bulk of the fluid (with probability 1- p att ). Dividing swarmers increase their chance of successful attachment by sticking a pilus on the surface followed by retraction before separation. Failure to stick a pilus leads to a release of the swarmer daughter in the bulk, where it is free to swim or be carried by flow. Full size image These findings demonstrate that a specific cell shape (curvature) can be beneficial in a specific environment (on surfaces with moderate flow). The curvature of C. crescentus causes cells to arc towards the surface in a flow field, thereby orienting and positioning its pili before retraction. The curved cell geometry also improves dispersal across flow, increasing microcolony size and surface coverage. We note that the distance between the stalked and the swarmer pole is shorter for a curved cell, potentially generating a more compact arrangement of attached cells compared with straight cells. When a microcolony reaches a critical density and size as a monolayer, newly divided cells can attach on top of neighbouring cells, thus generating multiple layers and tall colonies. Multiple layers build up more slowly and less robustly from the narrower and less dense creS microcolonies, which lead to reduced microcolony height compared with WT. Leveraging its shape and using multiple organelles for attachment and swimming, C. crescentus has evolved ways to balance sessile and planktonic lifestyles. Curvature, pili and the holdfast promote attachment and local development of multicellular structures, enabling robust colonization of nutrient-rich surfaces. Conversely, the flagellum favours dispersal via swimming, enabling exploration and colonization of distant environments. We speculate that C. crescentus could actively regulate the extent to which its daughter cells colonize a local environment or disperse to new environments. One mechanism for regulating surface attachment would be to increase the distance between the surface and the swarmer pole by lengthening the stalk. This mechanism could explain why C. crescentus cells markedly increase their stalk length when starved for phosphate [20] , thereby promoting cell dispersal upon nutrient stress. Our findings suggest that modulating the extent of cell curvature could also provide a mechanism to regulate the extent of daughter-cell attachment or dispersal. This hypothesis raises the possibility that C. crescentus could control the extent of dispersal by linking its metabolic state with curvature. We therefore suggest that cells could actively modulate curvature on metabolic perturbations such as nutrient state. For example, Caulobacter could increase the fraction of cells that locally attach when conditions are locally favourable by increasing the extent of curvature, or could increase the fraction of cells that disperse into the flow in times of stress by reducing the extent of curvature. One potential mechanism for coupling metabolic state to cell curvature is suggested by our laboratory’s previous finding that polymerization of the metabolic enzyme CTP synthetase reduces cell curvature in C. crescentus [21] . Investigation of the connection between the physiological state of C. crescentus , its curvature, CtpS assembly and cell dispersal will be a future extension of our work. We also note the alternative hypothesis that Caulobacter may have evolved a fixed curvature as part of a hard-wired bet-hedging strategy that maintains a constant attachment probability. C. crescentus maintains its curved shape using CreS, an intermediate filament-like protein that does not have homologues in bacteria outside the Caulobacter genus. This suggests that other curved bacteria evolved their curved shape independently. We also note that C. crescentus is atypical of other curved bacteria as it also possesses a polar stalk with a holdfast and divides asymmetrically. Consequently, the selective pressures that maintain cell curvature in other bacteria may be distinct from C. crescentus . For example, the pathogen Helicobacter pylori maintains its curvature (more precisely, its helical shape) in part by the action of several peptidoglycan remodelling proteins [22] . Moreover, H. pylori is found in the gastrointestinal, sometimes within a dense microbiota where flow is most likely weak and unsteady, and initial evidence shows that loss of curved shape affects its motility in gels [22] . Thus, it remains to be determined whether the benefit of curvature for surface colonization in flow for C. crescentus also benefits other bacteria with similar shapes. There are evolutionary implications to our finding that curved C. crescentus only exhibits a net surface colonization advantage in the moderate flow environments. Consistent with the hypothesis that curvature specifically provides a selective advantage in moderate flow environments, C. crescentus is a freshwater species found in ponds, lakes and streams. In these environments, it encounters a wide range of shear stresses that likely include niches with moderate shear stresses. For example, we anticipate that wall shear stress is negligible at the bed of a pond where fluid is nearly quiescent or within confined spaces such as small cracks or divots. In contrast, wall shear stress can reach values larger than 1 Pa on a meter-scale riverbed with currents generating a fluid velocity on the order of 1 m s −1 (ref. 23 ). As a means of comparison, we measured flow-dependent changes in the fitness advantage of curved C. crescentus within this naturally occurring range of surface shear stresses (0 to ~1 Pa). While C. crescentus and its closely related species Caulobacter maris and Maricaulis maris all harbour a polar stalk capped with a holdfast, C. crescentus is curved while C. maris and M. maris have straight rod morphologies [24] . Both of these straight species are found in marine environments [24] and are obligate aerobes, so they most likely develop as communities attached to particles carried by flow near the ocean’s surface, where oxygen concentration is sufficient to sustain their growth. There, they likely encounter a different hydrodynamic environment with permanently high shear stress generated by unsteady turbulent flow, possibly reducing any advantage of curvature. Future studies will help establish whether the difference in shear stresses encountered in the natural environments of these related species indeed underlies the differences in their cell shapes. The lack of a clear benefit for curvature in standard laboratory growth conditions highlights the importance of studying bacteria in environments that better reflect their natural habitats. Identifying the conditions in which the shapes of other bacterial species are advantageous may improve our understanding of bacterial ecology in addition to our understanding of the functions of individual cell shapes. Future engineering efforts will replicate ever more realistic growth environments, enabling us to decipher the selective benefits of specific cellular features as well as the functions of the vast number of genes that are maintained in bacterial genomes yet are fully dispensable in standard laboratory growth conditions [25] , [26] . Growth and media We used the freshwater isolate C. crescentus CB15 as parental strain [27] . Cells were grown at 30 °C in peptone-yeast extract (PYE) medium, supplemented with 5 μg ml −1 kanamycin if necessary. For selection of mutants and strains with constitutive expression of fluorescent proteins, we used PYE agar plates supplemented with 25 μg ml −1 kanamycin or 3% sucrose. We grew E. coli cells used to construct plasmids in liquid and agar LB plates supplemented with respectively 30 μg ml −1 and 50 μg ml −1 kanamycin. Strains and plasmids We list strains and plasmid used in this work in Supplementary Table 2 and primers in Supplementary Table 3 . We generated in-frame deletions of pilA and flgE genes by using the plasmid pNPTS138. In brief, we amplified 500 bp regions upstream and downstream the gene of interest. We assembled each pair of products by sewing PCR, digested, inserted the product into pNTPS138, and finally transformed into E. coli S17 electrocompetent cells. We then screened single colonies for correct insertion, which were then used as plasmid source for transformation in CB15. We prepared electrocompetent C. crescentus cells by pelletting 3 ml of overnight cultures of CB15 WT in PYE, washed them three times with 1 ml of ice-cold water and transformed with ~200 ng of plasmid before plating on PYE kanamycin plates. After about 48 h of incubation, we inoculated single colonies in plain PYE allowing for recombination and streaked for single colonies on sucrose plates. We finally screened for correct recombination by PCR and confirmed deletion by sequencing. To generate fluorescently labelled WT and creS strains, we fused mKate2 (red) and Venus (yellow) fluorescent proteins to a modified lac promoter for constitutive expression [28] . We ligated this insert obtained by sewing PCR in the integrating plasmid pXGFPC-2 digested with EcoRI and XmaI [29] . We transformed the construct into E. coli XL1 blue, purified plasmids with correct insertion and finally transformed into WT and creS CB15 as described above (without sucrose counter-selection) before selection on kanamycin. The resulting strains are constitutively expressing fluorescent proteins under lac promoter control integrated in the CB15 and CB15 creS chromosomes. Microfabrication of flow chambers We fabricated our flow chambers using standard soft lithography [30] . In brief, we fabricated molds by spinning single or double layers of photoresist (SU8 2010 and 2025, Microchem) on 3-inch silicon wafers. These were then exposed to UV light through a high-resolution photomask defining the microchannels and developed. After coating the resulting mold with a vapour of chlorotrimethylsilane (Sigma-Aldrich), we poured PDMS (sylgard 184, Dow Corning) on the wafer and baked the polymer at 75 °C on a hot plate for about 2 h. We then peeled off the cured PDMS slab, cut out individual chips and punched 1 mm access ports to the channel ends. We finally plasma bonded each PDMS chip to a #1.5 glass coverslip. C. crescentus growth in flow chambers We grew all cells to mid-log phase at 30 °C in plain PYE before injection in the flow chamber. For competition experiments between WT and creS mutant, we mixed equal volumes of cell suspensions at identical density and used both combinations of fluorescent proteins in parallel (WT-Venus competing against creS -mKate and inversely). We then injected the cell mixture in the microchannel by pipetting via the access holes. We controlled the initial density of sessile cells by varying the cell concentration of the suspension or the incubation time in the channel. For growth experiments and observation of microcolony formation, we immediately washed the channels with PYE after introduction of the cell mixture, thus keeping an initially low cell density. This allowed for visualization of single isolated colonies during long-term experiments. For single cell division time and attachment experiments, we incubated the cell suspension for 5 min in the channel to reach higher density, which allowed for measurement of division times and attachment events from a large number of cells. For all competition experiments, we used the two swapped combinations of fluorescent proteins for WT and creS to avoid any bias. For clarity, we present all fluorescent images in false color (red for creS and green for WT). We performed all growth in microchannels at room temperature. We then connected the inlet to a disposable sterile syringe filled with media and the outlet to a waste container via 1.09 mm outer diameter PEEK tubing and 27G sterile needles. We then mounted the chamber on the microscope stage. We generated flow with a syringe pump, and controlled flowrate (2.5 to 25 μl min −1 ) and used various channel dimensions (100 μm to 600 μm wide and 25 μm to 100 μm deep) to generate a wide range of flow speeds in the chamber. To describe the intensity of flow at the vicinity of the wall, we calculated wall shear stress σ from applied flow rate Q using the following equation: where w and h are respectively the channel width and depth and μ the viscosity of water. We performed most flow experiments at 0.23 Pa. We performed control experiments without flow in a glass bottom dish (Fluorodish, World Precision Instruments). We applied cells grown to mid-log phase to the glass dish and allowed for attachment for 5 min. We then rinsed the dish multiple times with 3 ml of plain PYE before starting time-lapse microscopy. Fluorescence microscopy We imaged cells growing in a microchannel on an inverted Nikon TiE microscope, equipped with 40x 0.95 N.A. Plan Apo and 100x 1.4 N.A Plan Apo objectives. We acquired images using an Andor Ixon3 EMCCD camera for z-stacks and Clara CCD camera for all other experiments. We controlled the microscope and image acquisition using Nikon NIS Elements software. To measure colony growth, we focused on single cells with × 40 magnification and acquired images every 20 or 30 min for 20 h to 48 h. To measure single-cell division and attachment events, we acquired images at × 100 magnification every 5 min for 14 h. We centred all images at the channel centreline. To visualize pilus retraction events, we imaged WT by phase contrast at 6 to 12 frames per minute. We obtained confocal images at the Princeton Confocal Facility on a Perkin Elmer spinning disk confocal equipped with solid state 488 nm and 560 nm laser illumination. Image analysis We analysed microscopy images using Matlab (the Mathworks). To generate spatial temporal diagrams and growth curves ( Fig. 2b,d ), we used a time-lapse image of a developing colony starting from a single cell. We subtracted background from each frame and integrated intensity over the whole frame or used the average pixel intensity in the direction of flow. We then normalized these data by the intensity of the single initial cell. To build the histogram of microcolony area ( Fig. 7b ), we generated a mask from fluorescence images by setting a threshold on intensity and counted features larger than 100 μm 2 (~50 cells). To measure doubling time, we measured the number of frames between two divisions of a surface associated cell from our × 100 high-resolution images. With the same data, we visually determined whether the daughter cell was attaching after separation (Fig. 4b). We also manually recorded the position of the attached daughter-cell pole relative to the mother cell-stalked pole in Fig. 6a . Confocal images were reconstructed into volume images and converted into Movies using NIS Elements (Nikon). We obtained side views of cells ( Fig. 4c ) by 3D-deconvolution of z-stacks (Autoquant module, MediaCybernetics) with slices spaced by 100 nm increments and orthogonal views were generated using imageJ. We measured the distance h between the swarmer pole and the surface by analysing similar z-stacks ( Fig. 4d and Supplementary Fig. 3 ): we first cropped z-stacks from single pre-divisional cells by selecting the ones that displayed a clear septum on fluorescence images, we then generated orthogonal views of these cells from which we could measure the distance from the pole to the surface (detected by labelling the stalks with wheat germ agglutinin—alexa fluor 488 conjugate, Molecular Probes). We similarly measured cell orientation angles ( Fig. 6b ) by generating orthogonal views, without selecting for pre-divisional cells. For creS , we measured the angle of the centreline of the cell body. For WT, we used the stalk and the base of the cell body as a guide for the orientation angle. To further assess the correlation between swarmer pole distance to the surface and attachment probability ( Supplementary Fig. 4 ), we calculated the distance h for a wide range of shear stresses using measurements of cell body orientation. We projected cells of typical dimension on the axis perpendicular to the surface to obtain, respectively, for creS and WT: where the length of the stalk L stalk is 0.5 μm, the length of the cell body L is 3 μm, the radius of curvature R is 3.5 μm. There is a critical angle below which the prediction for h WT is negative, that is, when the pole of the curved cell is in contact with the surface. In this range, we assume the cell is laying flat against the surface, so we use a typical cell half width (0.3 μm) as approximate value for h WT . How to cite this article: Persat, A. et al. The curved shape of Caulobacter crescentus enhances surface colonization in flow. Nat. Commun. 5:3824 doi: 10.1038/ncomms4824 (2014). Disclaimer The funders had no role in study design, data collection and analysis, decision to publish, or preparation of the manuscript.